A safe lithium mimetic for bipolar disorder Lithium is the most effective mood stabilizer for the treatment of bipolar disorder, but it is toxic at only twice the therapeutic dosage and has many undesirable side effects. It is likely that a small molecule could be found with lithium-like efficacy but without toxicity through target-based drug discovery; however, therapeutic target of lithium remains equivocal. Inositol monophosphatase is a possible target but no bioavailable inhibitors exist. Here we report that the antioxidant ebselen inhibits inositol monophosphatase and induces lithium-like effects on mouse behaviour, which are reversed with inositol, consistent with a mechanism involving inhibition of inositol recycling. Ebselen is part of the National Institutes of Health Clinical Collection, a chemical library of bioavailable drugs considered clinically safe but without proven use. Therefore, ebselen represents a lithium mimetic with the potential both to validate inositol monophosphatase inhibition as a treatment for bipolar disorder and to serve as a treatment itself. Bipolar disorder affects 1–3% of the population, and the most effective treatment for stabilizing mood is lithium [1] . Lithium is also the only agent that reduces suicidal thoughts and actions [2] . Unfortunately, lithium is toxic at only twice the therapeutic dosage and has many undesirable side effects, including weight gain, thirst, tremor and kidney damage [3] . To develop a lithium mimetic—ideally a drug with its therapeutic action but without its disadvantages—would require an understanding of lithium’s mechanism of action, which, even after six decades of use [4] , remains controversial [5] . Lithium displaces magnesium ions and inhibits at least 10 cellular targets, all of which are components of intracellular signalling pathways [5] . However, targets inhibited by lithium at therapeutically relevant concentrations (0.6–1 mM) narrows the targets to two: glycogen synthase kinase 3ß (ref. 6 ) and inositol monophosphatase (IMPase) [7] , [8] , [9] . Both putative targets have experimental evidence for and against them based on genetics and pharmacology [6] , [9] , [10] , [11] , [12] . In addition, several chemically distinct bipolar medications (lithium, valproic acid and carbamazapine) have a common mechanism of action affecting the inositol cycle [13] . Inhibition of IMPase by lithium led to Berridge’s ‘inositol depletion hypothesis’, which suggests that inositol 1-phosphate (Ins1P) is accumulated and inositol is depleted [7] . Given that in neurons regeneration of phosphatidylinositol 4,5-bisphosphate requires recycling of inositol from Ins1P, lithium dampens signalling in cells with overactive signalling through the pathways using a G-protein-coupled receptor linked to phospholipase C (ref. 7 ). IMPase remains a potential therapeutic target for bipolar disorder, but its validation requires small-molecule inhibitors. However, little progress has been made in regard to inhibitors since a large effort by Merck yielded a potent (IC 50 300 nM) antagonist (L-690,330), but neither it nor its esterified prodrug (L-690,488) was bioavailable [14] , [15] . We now report that ebselen inhibits IMPase and acts as a lithium mimetic in mouse models of bipolar disorder. Repurposing reveals ebselen as an inhibitor of IMPase To identify an inhibitor of IMPase, we expressed human IMPase in bacteria and used it in an assay to screen the NIH Clinical Collection provided through the National Institutes of Health Molecular Libraries Roadmap Initiative [16] . Compounds in this collection have a history of use in human clinical trials, are drug-like with known safety profiles and may even be appropriate for direct human use in new disease areas ( www.nihclinicalcollection.com ). A primary screen at 100 μM of each drug in the collection identified ebselen ( Fig. 1a ) as an inhibitor of IMPase, and we characterized it further with a full concentration–response curve ( Fig. 1b ). The potency of ebselen against IMPase (IC 50 1.5 μM) compared favourably with that of the known but poorly bioavailable inhibitor L-690,330 (ref. 14 ) (IC 50 0.3 μM) and was greater than that of lithium (IC 50 0.8 mM; Fig. 1b ). Importantly, the greater potency of ebselen for IMPase ( Fig. 1b ) compared with glycogen synthase kinase 3β ( Fig. 1c ) demonstrates selectivity, making ebselen of diagnostic use in determining the therapeutic potential of IMPase inhibition. 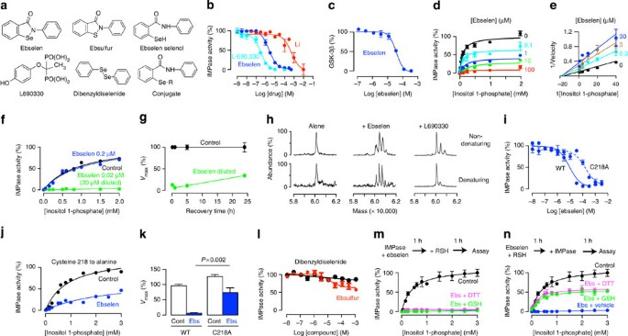Figure 1: Ebselen inhibits inositol monophosphatasein vitro. (a) Chemical structures. For the ebselen conjugate, R is GSH or another ebselen molecule. (b) Concentration–inhibition relationships for ebselen and known inhibitors of IMPase. Assay used expressed human IMPase. (c) Concentration–inhibition relationships for ebselen on glycogen synthase kinase 3β. (d,e) Effect of ebselen on the enzyme kinetics of IMPase shown as a Michaelis–Menten plot (d) or a Lineweaver–Burk plot (e). (f) Effect of dilution on inhibition of IMPase by ebselen (20 μM before and 0.2 μM after dilution). (g) Effect of recovery time after dilution on inhibition of IMPase by ebselen. (h) Mass spectrometry under mild denaturing and non-denaturing conditions of IMPase incubated with ebselen or L-690,330 (100 μM each). (i–k) Effect of mutation cysteine 218 to alanine on inhibition of IMPase by ebselen assessed by concentration–inhibition curves (i), Michaelis–Menten kinetics (ebselen 50 μM) (j) andVmax(k). Analysed by a pre-plannedt-test,n=6. (l) Concentration–response relationships for the sulphur analogue of ebselen and dibenzyldiselenide on IMPase. (m,n) Effect of disulphide reducing agents on inhibition of IMPase by ebselen (50 μM) with either post-incubation with GSH (1 mM) or DTT (50 mM) (m) or pre-incubation with 5 and 250 mM, respectively (n). All error bars represent s.e.m. Ebs, ebselen; WT, wild type. Figure 1: Ebselen inhibits inositol monophosphatase in vitro . ( a ) Chemical structures. For the ebselen conjugate, R is GSH or another ebselen molecule. ( b ) Concentration–inhibition relationships for ebselen and known inhibitors of IMPase. Assay used expressed human IMPase. ( c ) Concentration–inhibition relationships for ebselen on glycogen synthase kinase 3β. ( d , e ) Effect of ebselen on the enzyme kinetics of IMPase shown as a Michaelis–Menten plot ( d ) or a Lineweaver–Burk plot ( e ). ( f ) Effect of dilution on inhibition of IMPase by ebselen (20 μM before and 0.2 μM after dilution). ( g ) Effect of recovery time after dilution on inhibition of IMPase by ebselen. ( h ) Mass spectrometry under mild denaturing and non-denaturing conditions of IMPase incubated with ebselen or L-690,330 (100 μM each). ( i – k ) Effect of mutation cysteine 218 to alanine on inhibition of IMPase by ebselen assessed by concentration–inhibition curves ( i ), Michaelis–Menten kinetics (ebselen 50 μM) ( j ) and V max ( k ). Analysed by a pre-planned t -test, n =6. ( l ) Concentration–response relationships for the sulphur analogue of ebselen and dibenzyldiselenide on IMPase. ( m , n ) Effect of disulphide reducing agents on inhibition of IMPase by ebselen (50 μM) with either post-incubation with GSH (1 mM) or DTT (50 mM) ( m ) or pre-incubation with 5 and 250 mM, respectively ( n ). All error bars represent s.e.m. Ebs, ebselen; WT, wild type. Full size image Ebselen inhibition is irreversible and covalent As increasing concentrations of ebselen decreased V max with little effect on K m ( Fig. 1d ), the inhibition is not competitive [17] . Inhibition of IMPase by ebselen was not fully relieved by dilution (20–0.2 μM ebselen; Fig. 1f ), even after a time course for recovery extending to 25 h ( Fig. 1g ), thus indicating that inhibition is, for practical purposes, irreversible. A reversible inhibitor would lose potency upon dilution due to mass action promoting dissociation [17] . As irreversible inhibition often arises from covalent binding, we looked for direct evidence of ebselen binding to IMPase. Mass spectrometry revealed that a mixture of IMPase and ebselen formed complexes heavier than pure IMPase dimer by the mass of one or two ebselen molecules under both denaturing and non-denaturing conditions ( Fig. 1h ), supporting covalent binding and 1:1 stoichiometry per monomer. In contrast, a mixture of IMPase and the reversible inhibitor L-690,330 (ref. 14 ) formed heavier complexes under non-denaturing conditions, but not under denaturing conditions ( Fig. 1h ). Ebselen contains selenium ( Fig. 1a ), which can form a selenylsulfide (–Se–S–) bond [18] , [19] . For bovine IMPase, alkylation of cysteine 218 with the non-selective agent N -ethylmaleimide inhibited activity [20] . In bovine IMPase, cysteine 218 is near the active site residue aspartate 220, which is required for magnesium ion coordination and catalysis [20] . The position of this cysteine is conserved in both the mouse and human isoforms based on its crystal structure [21] . To test the importance of this cysteine in mediating ebselen inhibition, we constructed a human IMPase with a cysteine to alanine mutation (C218A). The C128A mutant was indeed less sensitive to ebselen inhibition, based on the increase in IC 50 for ebselen ( Fig. 1i ) and a smaller decrease in V max ( Fig. 1j ). Furthermore, an analogue ebselen in which the selenium is substituted with sulphur (ebsulfur; Fig. 1a ) weakly inhibited IMPase ( Fig. 1l ), whereas a selenium-containing compound with similar electrophilic reactivity (dibenzyldiselenide; Fig. 1a ) had no inhibitory effect ( Fig. 1l ). These data demonstrate that inhibition of IMPase by ebselen requires not just the presence of an electrophilic selenium atom but also an appropriate chemical scaffold. Unlike the case for most other proteins when covalently linked to ebselen [18] , [19] , [22] , inactivation of IMPase was not reversed by post-incubation with the sulfhydryl-reducing agents glutathione (GSH) and dithiothreitol (DTT) ( Fig. 1m ). Pre-incubation of ebselen with the reducing agents did, however, reduce inhibition ( Fig. 1n ) as described in detail below. Ebselen is pharmacologically active in the brain To determine whether ebselen can cross the blood–brain barrier and thus be pharmacologically active in mouse brain, as reported for rat [23] , we exploited the irreversible inhibition property of ebselen in an ex vivo method based on IMPase activity in brain homogenate ( Fig. 2a ). As the initial experiments that identified ebselen as an inhibitor used recombinant human IMPase ( Fig. 1b ), we first needed to ensure that recombinant mouse IMPase was enzymatically active. Recombinant mouse IMPase was inhibited by lithium, L-690,330 and ebselen ( Fig. 2b ). Having validated that ebselen inhibited the mouse form of IMPase, we demonstrated that in homogenates of mouse brain, IMPase activity was detectable and inhibited by lithium, L-690,330 and ebselen ( Fig. 2c ). In an ex vivo experiment, IMPase activity was measured in brain homogenates prepared at various times after intraperitoneal injection of ebselen ( Fig. 2a ) [24] . Over time, IMPase inhibition developed and then returned to control levels ( Fig. 2d ). Therefore, systemic administration of ebselen inhibits IMPase in mouse brain in whole animals. 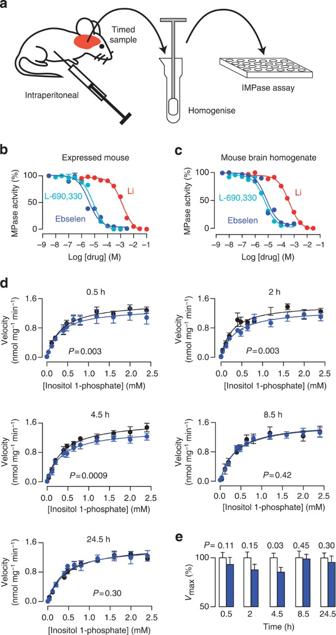Figure 2: Ebselen permeates the blood–brain barrier and inhibits endogenous inositol monophosphatase in mouse brain. (a) Schematic representation illustrating the experimental protocol for assessing IMPase inex vivoand brain homogenate experiments. Ebselen was injected at 10 mg kg−1. (b,c) Concentration–inhibition relationships for novel and known inhibitors of mouse IMPase expressed in bacteria (b) or present in homogenates from mouse brain (c). (d) Michaelis–Menten plots showing the effect of injected ebselen on IMPase inex vivobrain homogenate. Statistical significance was determined by a global fit of the Michaelis–Menten equation to the entire data set. (e) Effect of ebselen on theVmaxof IMPase over time after injection, analysed by pre-planned pairedt-test between the treatment nd control,n=5–6. All error bars represent s.e.m. Figure 2: Ebselen permeates the blood–brain barrier and inhibits endogenous inositol monophosphatase in mouse brain. ( a ) Schematic representation illustrating the experimental protocol for assessing IMPase in ex vivo and brain homogenate experiments. Ebselen was injected at 10 mg kg −1 . ( b , c ) Concentration–inhibition relationships for novel and known inhibitors of mouse IMPase expressed in bacteria ( b ) or present in homogenates from mouse brain ( c ). ( d ) Michaelis–Menten plots showing the effect of injected ebselen on IMPase in ex vivo brain homogenate. Statistical significance was determined by a global fit of the Michaelis–Menten equation to the entire data set. ( e ) Effect of ebselen on the V max of IMPase over time after injection, analysed by pre-planned paired t -test between the treatment nd control, n =5–6. All error bars represent s.e.m. Full size image That IMPase inhibition by ebselen was detected in the ex vivo experiments ( Fig. 2d ) is revealing in regard to the likely chemical form of ebselen in intact cells in vivo , as its selenium atom can exist in higher or lower oxidation states, and these have different reactivities [18] , [19] . Incubation of ebselen with reduced GSH forms ebselen–GSH selenenylsulphide, whereas incubation with DTT reduces ebselen to its selenol and diselenide ( Fig. 1a ) [18] , [19] . When we pre-incubated ebselen with these reducing agents, the reduced forms of ebselen (confirmed by mass spectrometry) were weaker inhibitors of IMPase ( Fig. 1n ), likely because they are less reactive with cysteines [18] . Therefore, to obtain inhibition of IMPase with ebselen in vivo , a fraction of ebselen must exist in a non-conjugated free form in the oxidation state shown in Fig. 1a , despite an intracellular environment with millimolar concentrations of reduced GSH [25] . Ebselen alters the function of the central nervous system To determine whether ebselen was affecting the function of the central nervous system, we investigated the effect of ebselen on the responses mediated by the serotonergic 5-HT 2 receptor [26] . In humans, lithium reduces phosphoinositide cycle-coupled 5-HT 2 receptor function [27] , and this may be linked to lithium’s antidepressant action. Lithium also reduces 5-HT 2 receptor function in mouse as modelled by a 5-HT 2 agonist-evoked head-twitch response [28] . This is mediated by the prefrontal cortex [29] , which is believed to be the target of lithium in the treatment of bipolar disorder [30] . Ebselen decreased 5-HT 2 agonist-induced head twitches in a dose-dependent manner ( Fig. 3a ), and this was associated with decreased expression of Arc mRNA (a molecular marker of neural activity [26] ) in the prefrontal cortex ( Fig. 3b ) and cingulate cortex ( Fig. 3c ). Thus, ebselen attenuates a cortically mediated 5-HT 2 receptor response that is linked to phosphoinositide turnover, as would be predicted for an inhibitor of IMPase. 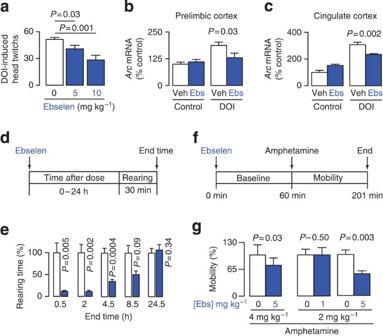Figure 3: Ebselen induces lithium-like behaviour. (a) Ebselen attenuates the head-twitch response induced by the 5-HT2Aagonist DOI (2 mg kg−1), analysed by pre-planned, one-tailedt-tests,n=6. (b,c) Ebselen (10 mg kg−1) attenuates the increase in the immediate-early geneArcmRNA induced by DOI (2 mg kg−1) in two cortical regions. Analysed by pre-planned, one-tailedt-tests,n=5–6. (d,f) Experimental protocols for assessing the effect of ebselen on behaviour in the open field test during exploratory activity (rearing,d) and amphetamine-induced hyperactivity (mobility,f). (e) Effect of ebselen (10 mg kg−1) on rearing over time, analysed by pre-planned pairedt-tests,n=5–6. (g) Effect of ebselen on mobility during amphetamine-induced hyperactivity, analysed by pre-planned pairedt-test,n=6–8. All error bars represent s.e.m. Ebs, ebselen. Figure 3: Ebselen induces lithium-like behaviour. ( a ) Ebselen attenuates the head-twitch response induced by the 5-HT 2A agonist DOI (2 mg kg −1 ), analysed by pre-planned, one-tailed t -tests, n =6. ( b , c ) Ebselen (10 mg kg −1 ) attenuates the increase in the immediate-early gene Arc mRNA induced by DOI (2 mg kg −1 ) in two cortical regions. Analysed by pre-planned, one-tailed t -tests, n =5–6. ( d , f ) Experimental protocols for assessing the effect of ebselen on behaviour in the open field test during exploratory activity (rearing, d ) and amphetamine-induced hyperactivity (mobility, f ). ( e ) Effect of ebselen (10 mg kg −1 ) on rearing over time, analysed by pre-planned paired t -tests, n =5–6. ( g ) Effect of ebselen on mobility during amphetamine-induced hyperactivity, analysed by pre-planned paired t -test, n =6–8. All error bars represent s.e.m. Ebs, ebselen. Full size image Ebselen exhibits lithium-like effects on behaviour Rodent behaviours are used to model bipolar disorder, and typically focus on either the manic or the depressive pole [31] . The ‘learned helplessness’ aspect of depression is often modelled with the forced swim test. In this model, ebselen has recently been shown to exhibit antidepressant action [32] . Given these findings, we investigated the effect of ebselen in lithium-sensitive mouse models of mania [33] . In the open field test ( Fig. 3d ), rearing was decreased by ebselen over time and then returned to baseline ( Fig. 3e ), a time course that paralleled that for IMPase inhibition in the ex vivo assay ( Fig. 2e ), as well as plasma ebselen concentrations in humans after oral administration [34] . Rearing is an exploratory behaviour that correlates with impulsivity [33] , which in turn correlates with suicidal thoughts and actions [35] . Mania has also been modelled by amphetamine-induced hyperactivity ( Fig. 3f ) [33] , [36] . Similarly to lithium [37] , ebselen reduced amphetamine-induced hyperactivity in a manner that depended on both the dose of amphetamine and the dose of ebselen ( Fig. 3g ), as is the case for lithium [37] . Baseline mobility was not significantly reduced (one-tailed, paired t -tests: amphetamine 2 mg kg −1 and ebselen 5 mg kg −1 , P =0.24; amphetamine 4 mg kg −1 and ebselen 5 mg kg −1 , P =0.08). Ebselen acts through inositol depletion Finally, if ebselen were mimicking lithium by inhibition of IMPase (and therefore inositol depletion), then one would expect ebselen’s effects to be circumvented by administration of exogenous inositol. This reversal is diagnostic of the ‘inositol depletion hypothesis’ if the addition of inositol re-establishes normal phosphatidylinositol 4,5-bisphosphate signalling [7] , [8] , [38] . We injected inositol intracerebroventricularly ( Fig. 4a ), and this reversed the effects of ebselen in models of both rearing ( Fig. 4b ) and amphetamine-induced mobility ( Fig. 4c ). Furthermore, mice injected intraperitoneally (i.p.) with ebselen showed a decrease in brain levels of inositol 1 h after administration ( Fig. 4d ), providing direct evidence for inositol depletion. In addition, these results are consistent with the known ability of inositol to reverse the behavioural effects of lithium [8] , [9] , [38] and support the inositol depletion hypothesis [7] . 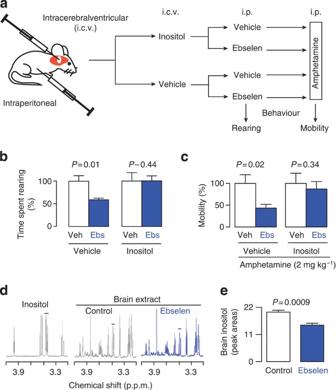Figure 4: The pharmacological effects of ebselen are mediated by inositol depletion. (a) Schematic representation outlining the experimental protocol used to investigate inositol reversal of behaviours induced by ebselen. Drugs were injected as follows: 1 μl of 0.5 M inositol, 5 mg kg−1ebselen and 2 mg kg−1amphetamine. (b) Effect of inositol on the ability of ebselen to attenuate rearing, analysed by pre-planned pairedt-tests between ebselen and control,n=4–6. (c) Effect of inositol on the ability of ebselen to attenuate amphetamine-induced hyperactivity (mobility) analysed by pre-planned pairedt-tests between ebselen and control,n=5–6. (d) Proton NMR spectra of authentic inositol and brain extracts from mice injected i.p. with either ebselen (10 mg kg−1) or hydroxypropyl β-cyclodextrin(4%w/v, control). (e) Effect of ebselen (10 mg kg−1) on inositol levels in mouse brain. Inositol was quantified by integration of the C1 and C3 peaks (indicated by the bar ind) and analysed by a pre-planned one-wayt-test between ebselen and control,n=4. All error bars represent s.e.m. Ebs, ebselen. Figure 4: The pharmacological effects of ebselen are mediated by inositol depletion. ( a ) Schematic representation outlining the experimental protocol used to investigate inositol reversal of behaviours induced by ebselen. Drugs were injected as follows: 1 μl of 0.5 M inositol, 5 mg kg −1 ebselen and 2 mg kg −1 amphetamine. ( b ) Effect of inositol on the ability of ebselen to attenuate rearing, analysed by pre-planned paired t -tests between ebselen and control, n =4–6. ( c ) Effect of inositol on the ability of ebselen to attenuate amphetamine-induced hyperactivity (mobility) analysed by pre-planned paired t -tests between ebselen and control, n =5–6. ( d ) Proton NMR spectra of authentic inositol and brain extracts from mice injected i.p. with either ebselen (10 mg kg −1 ) or hydroxypropyl β-cyclodextrin(4% w/v , control). ( e ) Effect of ebselen (10 mg kg −1 ) on inositol levels in mouse brain. Inositol was quantified by integration of the C1 and C3 peaks (indicated by the bar in d ) and analysed by a pre-planned one-way t -test between ebselen and control, n =4. All error bars represent s.e.m. Ebs, ebselen. Full size image Despite 60 years of use since its discovery as a mood stabilizer [4] , lithium remains the gold standard for the treatment of bipolar disorder [1] . Although combination therapy with an antidepressant is used to treat bipolar disorder, there is a risk of precipitating mania [39] . Uniquely, lithium is the only drug reported to reduce suicidal thoughts and behaviour [2] . Lithium is less than ideal, however, because of its undesirable side effects and toxicity. Therefore, there is a crucial need for drugs that are safe and efficacious for the treatment of bipolar disorder. Currently, drugs fail clinical trials primarily for reasons related to safety or efficacy [40] . Ebselen is known to be clinically safe [34] , [41] , and hence its efficacy should be tested. Ebselen exhibits lithium-like actions at many levels, including enzymatic, inositol recycling and animal behaviour, making it the best lithium mimetic reported to date [5] . In addition, ebselen is bioavailable, blood–brain barrier permeant and safer than lithium based on cellular toxicity [42] and phase 1–3 clinical trials [34] , [41] . Ebselen exhibits a polypharmacology profile ( http://mli.nih.gov/mli/mlp-probes/ ) that would be predicted to be beneficial in its role as a lithium mimetic because it directly inhibits the putative therapeutic targets of lithium, including IMPase and protein kinase C [43] , as well as being an antioxidant and inhibitor of cyclooxygenases that promotes neuronal survival [44] . Polypharmacology is much more common than previously appreciated [45] . Moreover, polypharmacology is now a desirable property [46] , [47] , for example, antipsychotics hitting multiple targets were more efficacious than drugs that were selective [48] . Inhibition of IMPase by ebselen is covalent and irreversible. Traditionally, covalent drugs have been disfavoured because of risks relating to immunogenicity [49] . However, covalent binding alone is not sufficient to cause problems [50] , and many marketed drugs act covalently [49] , demonstrating that such risks are compound specific. Importantly, ebselen has a good safety profile in all animal and human experiments reported to date [34] , [41] . Moreover, the irreversible action of ebelen on IMPase offers several advantages, as is the case for all irreversible drugs [49] , [51] , [52] . One advantage is that an irreversible inhibition cannot be overcome by accumulation of substrate. A second advantage is that irreversible inhibition can interact with pharmacokinetic effects to prolong ebselen’s duration of action and increase its selectivity for IMPase. After dosing, the decreasing concentration of ebselen will decrease its inhibition of all its reversible secondary targets. In contrast, IMPase will remain inhibited until new enzyme is synthesized. Such a scenario is known to be the case for many marketed drugs that are covalent and irreversible inhibitors, including the well-known drugs aspirin, clopidogrel and omeprazole [49] . There is an increasingly urgent need for new drugs for the treatment of mental illness, especially given that many large pharmaceutical companies have pulled out of these areas due to high costs and failure rates [39] , [53] , prompting speculation as to where new drugs will come from for treating disorders of the central nervous system [54] , [55] . Although there is no single solution, repurposing of drugs from their original use to a new use is being strongly promoted by government initiatives such as that announced by the NIH [16] , [56] , [57] . Given that ebselen has been in clinical trials [34] , [41] , ebselen offers all the promise of drug repurposing [58] . Recombinant inositol monophosphatase Murine MmImpa 1 and human HsImpa 1 were amplified from cDNA clones (IMAGE clones 6413389 and 3682657, respectively; Source Bioscience, Cambridge, UK). Cloning and protein expression were carried out as reported [21] , [59] . Semi-purified recombinant protein was obtained by heating lysed-cell supernatant (68 °C, 1 h) and centrifugation (30,000 g , 30 min, 4 °C). Cysteine 218 to alanine mutation in IMPase Site-directed mutagenesis of cysteine 218 was carried out using the Stratagene QuickChange kit. Protein was expressed as before, but without sorbitol and betaine. IMPase activity Phosphate hydrolysed from Ins1P was detected using the malachite green assay. For the in vitro assays, recombinant Hs IMPase (10 ng per well) or Mm IMPase (30 ng per well) was incubated (1 h, 37 °C) with Ins1P (1 mM) in 20 μl Tris buffer (50 mM Tris–HCl, 1 mM EGTA, 3 mM MgCl 2 , 150 mM KCl, 0.5 mg ml −1 BSA and 0.01% v/v Triton X pH 7.4). Absorbance was measured at 595 nm for samples and phosphate standards. For the ex vivo assays, brain homogenate (0.5 mg ml −1 ) was incubated (37 °C, 1 h) with Ins1P (0.1–2.4 mM) in the presence or absence of LiCl (30 mM) to determine IMPase-specific activity. Chemical library and screening The NIH Clinical Collection of 450 compounds was provided by the National Institute of Health [16] and purchased from BioFocus DPI. Compounds (100 μM) were screened at three concentrations of Ins1P. Initial hits were confirmed with concentration–inhibition curves spanning six orders of magnitude. Subsequent experiments used ebselen from Fisher Scientific. For compound screening, compound at 100 μM (in 0.2% v/v DMSO) was incubated with IMPase (10 min, room temperature) in buffer, before addition of Ins1P (1 mM) to a final volume of 20 μl, and further incubated (37 °C, 1 h). Phosphatase concentration was determined by the malachite green assay. LiCl and L-690,330 (Tocris) were used as positive controls. Reduced ebselen Ebselen (250 μM) was treated with 0.25 M DTT or 5 mM GSH; reduced ebselen (final concentration 50 μM) was incubated (1 h, room temperature) with Hs IMPase before addition of Ins1P (0.1–3 mM) and further incubation (1 h, 37 °C). Enzyme activity was determined by the malachite green assay. Testing for reversibility of drug inhibition Hs IMPase (1 μg per well) was incubated with 20 μM drug for varying times before dilution to 10 ng per well, addition of Ins1P and further incubation (1 h, 37 °C). Enzyme activity was determined by the malachite green assay. Selenyl–sulphur reversibility Conditions were as described above, except that 2 μl of reductant (50 mM DTT or 1 mM GSH) was added to each well, after incubation of IMPase with ebselen. Mass spectrometry IMPase (100 μM) was desalted using a Bio-Spin 6 Column (Bio-Rad) in 15 mM ammonium acetate (pH 7.5) and incubated (room temperature, 15 min) with 10 mM MgCl 2 before non-denaturing electrospray ionization mass spectrometry analysis (Q-TOF micro; Micromass). Data were processed with MASSLYNX 4.0 (Waters). To investigate IMPase ligand binding, mass spectrometry was used as described [60] , but with an additional mild denaturing step. Hs IMPase (100 μM) was incubated with 100 μM drug (10 min), then diluted (1:10) in 15 mM ammonium acetate buffer (pH 7.4) with 0.1% v/v formic acid. This solution was then subjected to mass spectrometry. Animals All studies used 20–25 g 10–12-week-old male C57Bl6 mice (Harlan Olac, UK). Mice were housed with 12 h light–dark cycles with free access to standard lab chow and water. The mice were acclimatised for a period of one week before any experiments were carried out. Experiments were carried out in accordance with UK Home Office Animals (Scientific Procedures) Act (1986) and associated code of practice guidelines. Animals were dosed intraperitoneally at 10 μl g −1 , unless otherwise specified. Lithium was dosed intraperitoneally at 67 μl g −1 . Ex vivo mouse brain homogenate Mice were injected with ebselen (10 mg kg −1 ) or vehicle (4% w/v hydroxypropyl β-cyclodextrin) and left for varying amounts of time before euthanization by cervical dislocation, or by CO 2 followed by cervical dislocation. Brains were removed and frozen on dry ice immediately. One hemisphere was homogenized using a Precellys 24-bead mill homogenizer (Stretton) and diluted in Tris buffer (50 mM Tris–HCl, 3 mM MgCl 2 , 150 mM KCl, 1 mM EGTA and 0.01% v/v Triton X pH 7.4) to a final concentration of 0.5 mg ml −1 . Ex vivo inositol measurement by nuclear magnetic resonance Mice were euthanized by cervical dislocation 1 h after administration of ebselen (10 mg kg −1 ) or vehicle (4% w/v hydroxypropyl β-cyclodextrin), then brains were extracted and frozen immediately on dry ice. Brains were weighed then homogenized using a Precellys 24-bead mill homogenizer (Stretton). Acetonitrile was added to homogenate (1:1 v / v ) to precipitate protein, the sample was centrifuged (13,000 g , 10 min) and the supernatant was prepared for NMR by lyophilization and reconstitution in D 2 O with 0.008% w/v 3-(trimethylsilyl)propionic 2233d acid sodium salt (600 mg ml −1 ). Amphetamine-induced hyperactivity Mice were treated with ebselen or vehicle and immediately placed in Linton AM1053 X, Y, Z IR Activity Monitor (San Diego Instruments) for 1 h to habituate. Mice were then injected with D -amphetamine/saline and returned to the cage, and activity was monitored for an additional 1 h. Rearing behaviour Mice were injected with ebselen (10 mg kg −1 ) or vehicle (4% w/v hydroxypropyl β-cyclodextrin) and left for varying amounts of time before being placed in the Linton AM1053 X, Y, Z IR Activity Monitor (San Diego Instruments) for 30 min while their activity was monitored. Rearing was measured by counting the number of beam breaks in upper grid. Intracerebroventricular injection of inositol Inositol reversal experiments were performed as described [38] . With mice under isoflurane-induced general anaesthesia, a guide cannula was stereotaxically implanted to 1 mm above the injection site in the lateral ventricle, and held in place with dental cement (Aqualox). Mice were left to recover for 7 days before behavioural studies were carried out. Inositol (5 or 1 μl of a supersaturated solution ≥278 mM) or control (0.9% w/v NaCl) was injected intracerebroventricularly, then 24 h later, amphetamine-induced hyperactivity was assessed as described above. Group means were compared with pre-planned t -tests, one-tailed or paired as appropriate. DOI-induced head twitches Mice were placed in an arena and left to acclimatize to the novel environment. After 1 h, they were injected with vehicle or ebselen (5 or 10 mg kg −1 ) followed 1 h later by the non-selective 5-HT 2A agonist 1-(2,5-dimethoxy-4 iodophenyl)-2-aminopropane (DOI, 2 mg kg −1 ). Head twitches were recorded 5 min after agonist injection for 15 min. Mice were constantly monitored by a video camera, and behavioural recordings were analysed offline independently by two observers who were blind to the treatment. In situ hybridization For quantification of Arc mRNA, brains were removed 1 h after the last injection of drug or vehicle and snap frozen in isopentane cooled by dry ice. Brain tissue sections (12 μm) were cut in a cryostat (−21 °C), thaw-mounted onto gelatine-subbed slides and stored (−80 °C), and then pretreated using standard methods. For in situ hybridization, oligonucleotides complimentary to Arc mRNA were 3′-tail labelled with [ 35 S]dATP and applied to each section in hybridization buffer (1 × 10 −6 cpm per section). After overnight incubation at 37 °C, sections were washed in buffer (150 mM NaCl and 15 mM sodium citrate, pH 7), first at 55 °C (3 × 20 min) and then at room temperature (2 × 60 min). Sections were then allowed to dry overnight and exposed to Kodak Biomax MR film (Sigma–Aldrich) for 7 days at room temperature. Films were developed and analysed with a computerized image analysis system using densitometric software (MCID, Linton, UK). Statistical analyses Means were compared with pre-planned t -tests (one-tailed or paired as appropriate) using GraphPad Prism software. All data are presented as mean±s.e.m. of the mean. How to cite this article: Singh, N. et al. A safe lithium mimetic for bipolar disorder. Nat. Commun. 4:1332 doi: 10.1038/ncomms2320 (2013).